Structural basis for oligomerization of auxin transcriptional regulators The plant hormone auxin is a key morphogenetic regulator acting from embryogenesis onwards. Transcriptional events in response to auxin are mediated by the auxin response factor (ARF) transcription factors and the Aux/IAA (IAA) transcriptional repressors. At low auxin concentrations, IAA repressors associate with ARF proteins and recruit corepressors that prevent auxin-induced gene expression. At higher auxin concentrations, IAAs are degraded and ARFs become free to regulate auxin-responsive genes. The interaction between ARFs and IAAs is thus central to auxin signalling and occurs through the highly conserved domain III/IV present in both types of proteins. Here, we report the crystal structure of ARF5 domain III/IV and reveal the molecular determinants of ARF–IAA interactions. We further provide evidence that ARFs have the potential to oligomerize, a property that could be important for gene regulation in response to auxin. Auxin is a key morphogenetic regulator involved in almost all aspects of plant development. In Arabidopsis thaliana , auxin-dependent gene regulation is mediated by one of the 23 members of the auxin response factors (ARF) family of transcription factors, which can either activate or repress transcription [1] , [2] . Interaction studies have shown that most of the 29 Aux/indole acetic acid (IAA) proteins are able to form complexes with ARF activators [2] , [3] and that IAAs mediate the recruitment of the TOPLESS corepressor [4] , thus acting as repressors of transcription of auxin-responsive genes. In contrast, very limited interactions occur between IAAs and ARF repressors [3] . When present, auxin promotes the ubiquitination and subsequent degradation of IAAs by the proteasome, thus releasing ARF activators from their repressive effect [1] . In this process, IAAs act as auxin coreceptors together with the transport inhibitor1 (TIR1) or auxin-signalling F-box protein (AFB) F-box proteins, which belong to the SCF E3 ubiquitin ligase complex responsible for catalyzing the degradation of the IAAs [5] , [6] . Protein–protein interactions between ARF and IAA proteins are central to auxin signalling and occur through a conserved region called domain III/IV [7] . Based mainly on yeast two-hybrid assays (Y2H) and on protoplast transfection assays, the domain III/IV has been proposed to mediate both the formation of ARF or IAA homodimers as well as ARF–IAA heterodimers [2] . We report here the crystal structure of ARF5 domain III/IV and identify the molecular determinants controlling interactions between ARFs and IAAs. We further demonstrate that ARFs and IAAs can oligomerize, a property that could be crucial for gene regulation in response to auxin. Structure determination To understand the molecular determinants of the interactions between auxin signalling components, we solved the crystal structure of the domain III/IV of ARF5 (III/IV ARF5 ) ( Fig. 1a–c ), an ARF activator essential from embryogenesis onward and also known as MONOPTEROS [8] . We found that this domain shows strong structural similarity with an A/B PB1 domain ( Fig. 1d ) as previously proposed based on homology modelling [7] , but with an additional long C-terminal α-helix. In the crystal, III/IV ARF5 form oligomers in which monomers interact with each other in a head-to-tail manner, with each monomer contacting its neighbours through two charged interfaces: one generally positive (+ face) and another generally negative (− face) ( Fig. 1b,c,e ). K797 from the positive side of one monomer interacts with D847, E849 and D851 of the OPCA motif of another monomer as described previously in other A/B PB1 domains [9] . However, additional polar and hydrogen interactions are found between R793, T794, Q799, G805, R806 and S807 of the positive face and D858, E862, D851, V852, D857 and D857 of the negative face, respectively ( Fig. 1b,e and f ; Supplementary Fig. 1 ). 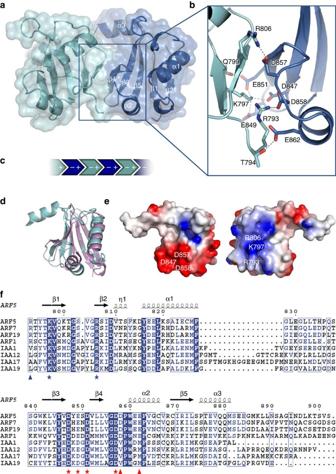Figure 1: Structural determinants for III/IVARF5oligomerization. (a) Structure of two III/IVARF5interacting monomers. Cartoon and surface representation showing one III/IVARF5monomer (in cyan) interacting with another one (in blue). In the crystal, each monomer interacts with another monomer in a head-to-tail manner. (b) Main interactions at the III/IVARF5interface. R793, T794, K797, Q799 and R806 of the positive face interact with D847, E849, D851, D857, D858 and E862 of the negative face. Note that the electron density for R793 was relatively poor in some subunits. (c) Cartoon showing the head-to-tail interactions of III/IVARF5in the crystal. (d) The PB1 domain of PAR6 (ref.26) (1WMH; RMSD of 2.2 Å for 71 Cα) was identified as the closest match to the ARF5 III/IV domain using Dali27. PAR6 (inpink) is shown structurally aligned to ARF5 (in cyan). Note that an ARF5 specific C-terminal helix extends from the main PB1 domain. (e) Electrostatic surfaces showing that ARF5 exhibits a generally positively charged (in blue) and a generally negatively charged (in red) interface as shown using DELPHI28and PyMOL29. (f) Alignment of ARF and IAA fromA. thalianausing ESPript30.Blueandredasterisks indicate conserved residues of the positive and negative face, respectively.Blueandredtriangles show conserved residues of the positive and negative face found only in the ARF family. Figure 1: Structural determinants for III/IV ARF5 oligomerization. ( a ) Structure of two III/IV ARF5 interacting monomers. Cartoon and surface representation showing one III/IV ARF5 monomer (in cyan) interacting with another one (in blue). In the crystal, each monomer interacts with another monomer in a head-to-tail manner. ( b ) Main interactions at the III/IV ARF5 interface. R793, T794, K797, Q799 and R806 of the positive face interact with D847, E849, D851, D857, D858 and E862 of the negative face. Note that the electron density for R793 was relatively poor in some subunits. ( c ) Cartoon showing the head-to-tail interactions of III/IV ARF5 in the crystal. ( d ) The PB1 domain of PAR6 (ref. 26 ) (1WMH; RMSD of 2.2 Å for 71 Cα) was identified as the closest match to the ARF5 III/IV domain using Dali [27] . PAR6 (in pink ) is shown structurally aligned to ARF5 (in cyan). Note that an ARF5 specific C-terminal helix extends from the main PB1 domain. ( e ) Electrostatic surfaces showing that ARF5 exhibits a generally positively charged (in blue) and a generally negatively charged (in red) interface as shown using DELPHI [28] and PyMOL [29] . ( f ) Alignment of ARF and IAA from A. thaliana using ESPript [30] . Blue and red asterisks indicate conserved residues of the positive and negative face, respectively. Blue and red triangles show conserved residues of the positive and negative face found only in the ARF family. Full size image In vitro validation of ARF and IAA interaction surfaces To test the interactions observed in the crystal in solution, we performed site-specific mutagenesis of key III/IV ARF5 interface residues and analysed the resulting complexes using size exclusion chromatography (SEC). III/IV ARF5 (hereafter referred to as ARF5) elutes as an oligomer of about 10 molecules with an asymmetric elution peak suggesting variability in the number of monomers ( Fig. 2 ). Simultaneous mutation of the positive (K797S) and the negative faces (D857S; mutant ARF5m3) as well as mutations affecting only the positive face (R793S-K797S-R806S, ARF5m1) or the negative face (D847S-D857S-D858S, ARF5m2) abolished ARF5 oligomerization leading to ARF5 monomers with a small proportion of ARF5 dimers ( Fig. 2 ). We thus confirmed that ARF5 can form oligomers and that the observed interaction surface occurs in solution. 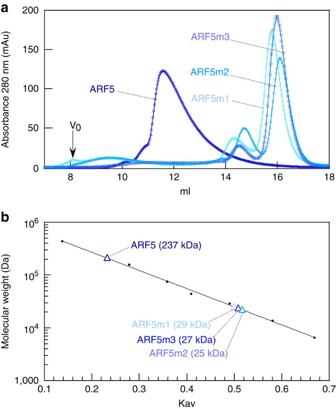Figure 2: Analysis of ARF5 domain III/IV oligomerization. (a) SEC analysis showing that the wild-type ARF5 is eluted as a large oligomer and that mutation on the positive face (ARF5m1), the negative face (ARF5m2) or both faces (ARF5m3) leads to a monomer with a small proportion of dimer. (b) Calibration curve used to determine the apparent molecular weight of proteins shown ina. Isolated domains III/IV were used and fused to a 6his-tag. v0 indicates the void volume of column. III/IVARFproteins and calibration standards were loaded in the same buffer (see Methods). Figure 2: Analysis of ARF5 domain III/IV oligomerization. ( a ) SEC analysis showing that the wild-type ARF5 is eluted as a large oligomer and that mutation on the positive face (ARF5m1), the negative face (ARF5m2) or both faces (ARF5m3) leads to a monomer with a small proportion of dimer. ( b ) Calibration curve used to determine the apparent molecular weight of proteins shown in a . Isolated domains III/IV were used and fused to a 6his-tag. v0 indicates the void volume of column. III/IV ARF proteins and calibration standards were loaded in the same buffer (see Methods). Full size image Many amino acids involved in ARF5 oligomerization are also conserved in IAA proteins ( Fig. 1f ; Supplementary Fig. 1 ), suggesting that IAA proteins might assemble into an oligomer using the same mode as ARFs. We tested this hypothesis for the domain III/IV of IAA12 (ref. 10 ). Because this domain has a marked tendency to aggregate and precipitate in most buffers, we had to formulate a solubilization buffer, which reduced its aggregation. In this buffer, we found that wild-type IAA12 formed a trimer, whereas IAA12 mutants affected on the positive (K128S-R138S, IAA12m1), the negative (D189S-D199S, IAA12m2) or both faces (K128S-D199S, IAA12m3) became monomeric ( Fig. 3a–c ). As observed for ARF5, the asymmetric shape of the elution peak of IAA12 indicates a mix of oligomers of different sizes. These results suggested that the ARF interaction mode also applied to IAA proteins. 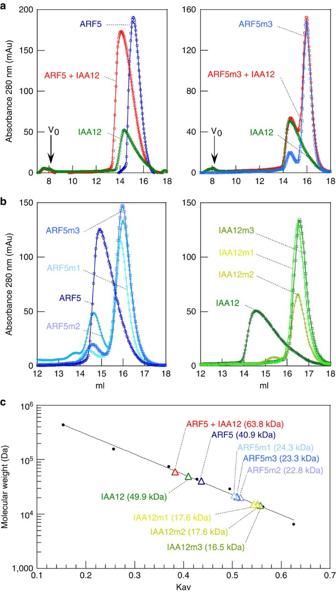Figure 3: Analysis of ARF–IAA interactions using gel-filtration experiments. (a) SEC analysis of ARF5 (blue), IAA12 (green) or both proteins mixed (red). By contrast to the wild-type ARF5, the ARF5m3 double mutant is unable to interact with IAA12 (right). (b) SEC analysis of ARF5 (left) and IAA12 proteins (right). Oligomerization of ARF5 and IAA12 is impaired by mutation of the positive face (ARF5m1, IAA12m1), the negative face (ARF5m2, IAA12m2) or both faces (ARF5m3, IAA12 m3). (c) Calibration curve used to estimate apparent molecular weight of proteins presented inaandb. According to this curve, ARF5 is eluted as a dimer, IAA12 as a trimer and ARF5m1, ARF5m2, ARF5m3, IAA12m1, IAA12m2 and IAA12m3 are eluted as monomers. Isolated domains III/IV were used for ARF and IAA proteins. All proteins (ARF, IAA and calibration standards) were loaded in the solubilization buffer (see Methods). Figure 3: Analysis of ARF–IAA interactions using gel-filtration experiments. ( a ) SEC analysis of ARF5 (blue), IAA12 (green) or both proteins mixed (red). By contrast to the wild-type ARF5, the ARF5m3 double mutant is unable to interact with IAA12 (right). ( b ) SEC analysis of ARF5 (left) and IAA12 proteins (right). Oligomerization of ARF5 and IAA12 is impaired by mutation of the positive face (ARF5m1, IAA12m1), the negative face (ARF5m2, IAA12m2) or both faces (ARF5m3, IAA12 m3). ( c ) Calibration curve used to estimate apparent molecular weight of proteins presented in a and b . According to this curve, ARF5 is eluted as a dimer, IAA12 as a trimer and ARF5m1, ARF5m2, ARF5m3, IAA12m1, IAA12m2 and IAA12m3 are eluted as monomers. Isolated domains III/IV were used for ARF and IAA proteins. All proteins (ARF, IAA and calibration standards) were loaded in the solubilization buffer (see Methods). Full size image We next explored the molecular basis of the interaction between ARF5 and its interacting partner IAA12 (also known as BODENLOS; ref. 10 ) in the solubilization buffer that allows both protein domains to be soluble but reduces ARF5 complexes to dimers ( Fig. 3b,c ). Using SEC, we found that ARF5 and IAA12 could interact and that their interaction was abolished by mutating the + and – faces of ARF5 ( Fig. 3a,c ). Directionality of the ARF5-IAA12 interactions As ARFs and IAAs possess A/B PB1-like domains, heterodimerization could formally occur through either face: the ARF + face with the IAA − face and the ARF − face with the IAA + face. We thus assayed the directionality of these interactions. To avoid homo-oligomer interference and specifically observe ARF–IAA contact, we used pull-down assays on purified domain and Y2H assays. Both pull-down assays (flowing IAA12 onto immobilized ARF5 and vice versa) and Y2H assays confirmed that wild-type IAA12 and ARF5 could interact and that this interaction was strongly reduced when one of the two partners was mutated on both the + and − faces ( Fig. 4a–c ). To test whether each face of IAA12 could be involved in interaction with ARF5, we mutated them individually. In pull-down assays, disrupting the IAA12 positive face (IAA12m1) or its negative face (IAA12m2), reduced complex formation without abolishing it ( Fig. 4b ). Similarly, IAA12 proteins mutated on a single face were still able to interact with ARF5 in Y2H assays ( Fig. 4c ). Taken together, these data strongly suggest that IAA12 can indeed interact with ARF5 both via its negative and positive faces. 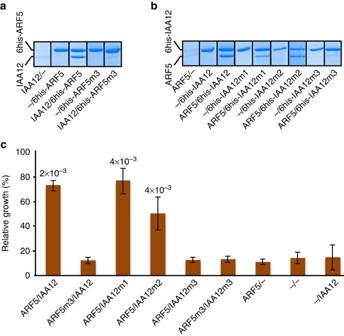Figure 4: Analysis of ARF–IAA interactions using pull-down and yeast two-hybrid assays. (a) Pull-down assays showing that 6his-ARF5 bound to a Ni-Sepharose column interacts with free IAA12 and that this interaction is impaired with 6his-ARF5m3 mutated on both faces. SDS–PAGEs show the proteins eluted from the column after initial binding of 6his-ARF5, addition of untagged IAA12 and washing. (b) Pull-down assays showing that free ARF5 still interacts with 6his-IAA12m1 mutated on its positive face and with 6his-IAA12m2 mutated on its negative face. The double mutant altered on both faces (6his-IAA12m3) lost its capacity to interact with ARF5. SDS–PAGE shows the proteins eluted after initial binding of 6his-IAA12 to the column, addition of untagged ARF5 and washing. Full images of protein gels are shown asSupplementary Figure 3. Isolated domains III/IV were used for ARF5 and IAA12 proteins. (c) Y2H experiments showing that wild-type ARF5 can interact via both faces of IAA12.P-values from one-sided Mann–WhitneyU-test (n=4 for all experiments) by comparison with the results obtained with the two empty vectors (−/−) are indicated. Error bars represent s.d. Isolated domains III/IV were used for ARF5 and full-length proteins for IAA12. Figure 4: Analysis of ARF–IAA interactions using pull-down and yeast two-hybrid assays. ( a ) Pull-down assays showing that 6his-ARF5 bound to a Ni-Sepharose column interacts with free IAA12 and that this interaction is impaired with 6his-ARF5m3 mutated on both faces. SDS–PAGEs show the proteins eluted from the column after initial binding of 6his-ARF5, addition of untagged IAA12 and washing. ( b ) Pull-down assays showing that free ARF5 still interacts with 6his-IAA12m1 mutated on its positive face and with 6his-IAA12m2 mutated on its negative face. The double mutant altered on both faces (6his-IAA12m3) lost its capacity to interact with ARF5. SDS–PAGE shows the proteins eluted after initial binding of 6his-IAA12 to the column, addition of untagged ARF5 and washing. Full images of protein gels are shown as Supplementary Figure 3 . Isolated domains III/IV were used for ARF5 and IAA12 proteins. ( c ) Y2H experiments showing that wild-type ARF5 can interact via both faces of IAA12. P -values from one-sided Mann–Whitney U -test ( n =4 for all experiments) by comparison with the results obtained with the two empty vectors (−/−) are indicated. Error bars represent s.d. Isolated domains III/IV were used for ARF5 and full-length proteins for IAA12. Full size image In planta validation of interaction surfaces To validate our findings in vivo , we tested the effect of wild-type and mutant ARF7 (another ARF activator), IAA17 and IAA19 on the expression of the DR5::GUS auxin-inducible synthetic reporter in plant protoplasts ( Fig. 5 ). In this system, auxin-dependent gene induction is activated by ARF7 and repressed by IAA17 and IAA19 (ref. 11 ). We found that ARF7 became able to induce DR5 expression independently of auxin only when mutated on both faces, indicating that IAA proteins can perform their repressive effect by targeting both faces of ARF7 ( Fig. 5a ). Furthermore, we observed that the repressive capacities of IAA17 and IAA19 were most lowered by mutations on both faces (IAA17/19m3) compared with mutations on a single face (IAA17/19m1 and IAA17/19m2; Fig. 5b ). Note that the repressive capacities of IAAs are not entirely lost when mutated on both faces (IAA17/19m3), possibly due to a residual interaction with ARF7. Consistent with this idea, a slight capacity to dimerize is still observed with ARF5 mutated on both faces (ARF5m3; Fig. 2a ). In conclusion, these results establish the biological relevance of the interface identified in the ARF5 structure and confirm that IAAs can interact with both sides of ARFs in vivo . 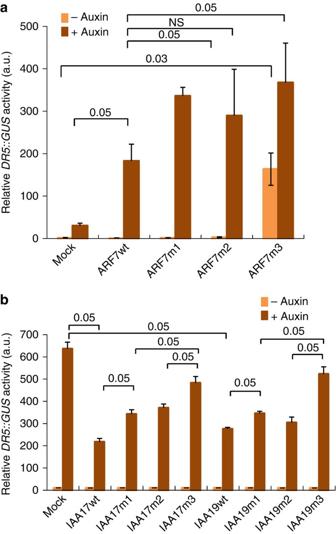Figure 5:In plantavalidation of ARF–IAA interactions. (a,b) Signalling activity of wild-type and mutant ARF7, IAA17 and IAA19 inArabidopsis thalianaprotoplasts expressing the auxin-inducible DR5::GUS reporter. (a) Comparison of the capacity of the wild-type ARF7 (ARF7wt) and of mutant forms affected on the positive face (K1042A-R1051A: ARF7m1), on the negative face (D1092A-D1096A-D1102A-D1103A: ARF7m2) or on both (K1042A-D1092A-D1096A-D1102A-D1103A: ARF7m3) to induce auxin-signalling activity in absence (IAA−) or presence (IAA+) of auxin. ARF7 wild-type and mutant forms all significantly increase auxin-induced transcription, as monitored byDR5::GUS. However, only ARF7m3 can increase the transcription of DR5::GUS in the absence of auxin. (b) Comparison of the capacity of the wild-type IAA17 and IAA19 (IAA17/19wt) and mutant forms affected on the positive face (K114A: IAA17m1; K100A: IAA19m1), on the negative face (D183A-D187A: IAA17m2; D154A-D158A: IAA19m2) or on both (K114A-D183A-D187A: IAA17m3; K100A-D154A-D158A: IAA19m3) to repress auxin-signalling activity in absence (IAA−) or presence (IAA+) of auxin. Expression of IAA17 or IAA19 reduces the induction of DR5::GUS in response to auxin, indicating repression of auxin signalling by the IAA proteins. The repressive capacities are slightly reduced by mutations affecting a single IAA face (m1 and m2) and more importantly affected by mutations affecting both faces (m3) for both IAA17 and IAA19.P-values from one-sided Mann–WhitneyU-test (n=3 for all experiments). Error bars represent s.d. Figure 5: In planta validation of ARF–IAA interactions. ( a , b ) Signalling activity of wild-type and mutant ARF7, IAA17 and IAA19 in Arabidopsis thaliana protoplasts expressing the auxin-inducible DR5::GUS reporter. ( a ) Comparison of the capacity of the wild-type ARF7 (ARF7wt) and of mutant forms affected on the positive face (K1042A-R1051A: ARF7m1), on the negative face (D1092A-D1096A-D1102A-D1103A: ARF7m2) or on both (K1042A-D1092A-D1096A-D1102A-D1103A: ARF7m3) to induce auxin-signalling activity in absence (IAA−) or presence (IAA+) of auxin. ARF7 wild-type and mutant forms all significantly increase auxin-induced transcription, as monitored by DR5::GUS . However, only ARF7m3 can increase the transcription of DR5::GUS in the absence of auxin. ( b ) Comparison of the capacity of the wild-type IAA17 and IAA19 (IAA17/19wt) and mutant forms affected on the positive face (K114A: IAA17m1; K100A: IAA19m1), on the negative face (D183A-D187A: IAA17m2; D154A-D158A: IAA19m2) or on both (K114A-D183A-D187A: IAA17m3; K100A-D154A-D158A: IAA19m3) to repress auxin-signalling activity in absence (IAA−) or presence (IAA+) of auxin. Expression of IAA17 or IAA19 reduces the induction of DR5::GUS in response to auxin, indicating repression of auxin signalling by the IAA proteins. The repressive capacities are slightly reduced by mutations affecting a single IAA face (m1 and m2) and more importantly affected by mutations affecting both faces (m3) for both IAA17 and IAA19. P -values from one-sided Mann–Whitney U -test ( n =3 for all experiments). Error bars represent s.d. Full size image Taken together, our results have several important functional implications. It has been recently shown that the ARF5 DNA-binding domain possess a dimerization motif [12] . However, the III/IV ARF5 domain head-to-tail mode of interaction observed in the crystal and the analysis of III/IV ARF5 behaviour in solution show that the domain III/IV has the capacity to mediate more than just dimerization and might allow ARF proteins to oligomerize. While it remains to be established whether ARF full-length proteins indeed form oligomers in planta , this property could be critical for their DNA-binding capacity. Indeed, transcription factor oligomerization is a common mechanism allowing cooperative binding to multiple cis -elements, a property central to networks involving developmental switches [13] that could be relevant for cell-fate decisions in response to auxin. By interacting with both faces of ARF monomers, IAA might weaken the cooperativity of ARF oligomer DNA binding ( Fig. 6 ). Consistent with this idea, ARF5 DNA binding was shown to increase upon auxin application in vivo [14] , an observation that cannot be easily reconciled with current models of auxin action [1] and could be due to the ability of the IAA protein to cooperatively reduce ARF DNA binding. Also, it was shown that ARF5 lacking domain III/IV has a reduced capacity to bind DNA in vitro that can be compensated by antibody-induced dimerization [15] again suggesting that domain III/IV might contribute to DNA binding. While the combinatorial specificity of ARF and Aux/IAA interaction is extremely complex [3] , our data thus provide a structural framework with which to further study the intricate pattern of ARF and Aux/IAA interactions and their impact on the dynamics of auxin-induced signalling activity ( Fig. 6 ). 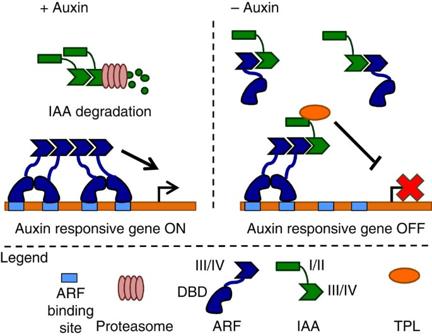Figure 6: Schematic model for auxin transcriptional components. Cartoon representing the putative role of domain III/IV from ARF and IAA proteins in auxin signalling. We speculate that IAA might perturb ARF DNA binding by decreasing its oligomerization. TPL, TOPLESS corepressor; DBD, DNA binding domain. Figure 6: Schematic model for auxin transcriptional components. Cartoon representing the putative role of domain III/IV from ARF and IAA proteins in auxin signalling. We speculate that IAA might perturb ARF DNA binding by decreasing its oligomerization. TPL, TOPLESS corepressor; DBD, DNA binding domain. Full size image ARF and Aux/IAA coding sequences and cloning Wild-type full-length coding sequences (CDS) for ARF5 and IAA12 (ref. 3 ) were used as matrix for amplification. All oligonucleotides used for this study are listed in Supplementary Table 1 . A set of mutated sequences of the conserved domain III/IV of ARF5 (ARF5 CTD: S779 to S902) and of the full-length IAA12 CDS were synthesized (GeneCust): ARF5m1 (R793S-K797S-R806S), ARF5m2 (D847S-D857S-D858S), ARF5m3 (K797S-D857S), IAA12m1 (K128S-R138S), IAA12m2 (D189S-D199S) and IAA12m3 (K128S-D199S) from which the conserved domain III/IV was amplified using specific primers. For expression and purification of proteins, the domains III/IV of wild-type and mutant ARF5 and IAA12 (S779 to S902 for ARF5, L124 to V239 for IAA12) were cloned into the expression vector pETM-11 (ref. 16 ) containing a six-histidine tag and TEV-protease cleavage site sequences, positioned at the N-terminus of the recombinant proteins. For the Y2H tests, wild-type and mutant ARF5 domain III/IV (S779 to S902) and full-length IAA12 CDS were inserted by gateway cloning (LR reaction) following the manufacturer instructions (Invitrogen) in pACT2-based vector (downstream of Gal4-AD) and a pGBKT7-based vector for the ARFs (downstream of Gal4-BD) [3] . pUC19 vectors containing full-length ARF7, IAA17 and IAA19 cloned downstream of the 35S constitutive promoter and in which all of the constructs had an N-terminal HA tag were used for the protoplast assays. The following mutated versions of the proteins were obtained using the QuickChange site-directed mutagenesis kit (Stratagene): ARF7m1 (K1042A-R1051A), ARF7m2 (D1092A-D1096A-D1102A-D1103A), ARF7m3 (K1042A-D1092A-D1096A-D1102A-D1103A), IAA17m1 (K114A), IAA17m2 (D183A-D187A), IAA17m3 (K114A-D183A-D187A), IAA19m1 (K100A), IAA19m2 (D154A-D158A) and IAA19m3 (K100A-D154A-D158A). IAA17 and IAA19 are mutated in their domain II to create stabilized versions of these proteins [17] . Expression and purification of recombinant proteins Wild-type and mutant ARF5 and IAA12 III/IV domains were expressed using Escherichia coli strain Rosetta2 (DE3; Novagen, Darmstadt, Germany). After induction by 0.4 mM isopropyl β-D-1-thiogalactopyranoside (IPTG), cells were grown overnight at 17 °C. For cell lysis, the pellet of 500 ml culture was sonicated in 50 ml lysis buffer A (20 mM Tris pH 8.2, 1 mM tris (2-carboxyethyl)phosphine) (TCEP) for ARF5 and lysis buffer B (200 mM N -cyclohexyl-3-aminopropanesulfonic acid (CAPS) pH 10.5, 1 M NaCl, 1 mM TCEP) for IAA12 (in both cases, buffer A and B were supplemented with one protease inhibitor cocktail tablet complete EDTA-free (Roche, Meylan, France). After sonication, the solutions were centrifuged for 30 min at 13,000 g . The clear supernatant was loaded on 2 ml Ni-Sepharose High-Performance resin (GE Healthcare, Uppsala, Sweden) column. The resin was washed with 10 column volumes of buffer A for ARF5 or buffer B for IAA12 complemented with 30 mM imidazole. The recombinant proteins of interest ARF5 and IAA12 were eluted with buffer A and buffer B, respectively, complemented with 300 mM imidazole. For crystallization and some pull-down and SEC experiments, the His-tagged proteins were cleaved by the TEV protease and loaded to a second Ni-Sepharose High-Performance resin to remove the His-tag and the TEV protease. For crystallization, ARF5 was further purified on a Hi-load Superdex-200 16/60 prep grade column (GE Healthcare) equilibrated with buffer A. Purified 6his-ARF5 (17 kDa), 6his-IAA12 (16.5 kDa), cleaved ARF5 (14 kDa) and IAA12 (13.5 kDa) are shown in Supplementary Fig. 2 . SEC Apparent molecular weight of 6his-ARF5, 6his-ARF5m1, 6his-ARF5m2 and 6his-ARF5m3 was determined in buffer A supplemented with NaCl 100 mM on a Superdex-200 10/300GL column (GE Healthcare) calibrated with protein standards (GE Healthcare: Ferritin, 440 kDa; Aldolase, 158 kDa; Conalbumin, 75 kDa; Ovalbumin, 44 kDa, Carbonic anhydrase, 29 kDa; Ribonuclease A, 13.7 kDa; Aprotinin 6.5 kDa) ( Fig. 3b ) and using the equation MW=1.3196 × 10 6 × e (−7,9282 × Kav) (where MW=apparent molecular weight, Kav=(ve−v0)/(vc−v0); ve=elution volume of the protein, v0=void volume of the column (8.05 ml), vc=total volume of the column (24 ml)). ARF5 elutes as an oligomer with an apparent molecular weight (188 kDa) similar to 6his-ARF5 showing that the presence of the 6his-tag does not alter the oligomerization. Apparent molecular weight of ARF5 and IAA12 alone or in complex was also determined in the solubilization buffer C (10 mM Tris-HCl, CAPS, 100 mM pH 10.2, NaCl 0.5 M and 1 mM TCEP) allowing manipulation of both ARF5 and IAA12. Experiments were done on the Superdex-200 10/300GL column calibrated with the protein standards (GE Healthcare) in the solubilization buffer and using the equation MW=1.6335 × 10 6 × e (−8.5451 × Kav) (void volume of the column=8.05 ml) ( Fig. 4c ). For both buffers, 160 μg of protein (6his-ARF5, IAA12, standard proteins) in a final volume of 100 μl were injected on the column. Pull-down experiments The solubilization buffer allowing manipulation of both ARF5 and IAA12 was used for the pull-down experiments. One hundred and sixty μg of 6his-tagged-proteins (adjusted to 100 μl with buffer C (see above) were loaded on 50 μl of Ni-Sepharose High-Performance resin (GE Healthcare, Uppsala, Sweden). After washing the resin with buffer C supplemented with 30 mM imidazole, the untagged ARF5 or IAA12 was loaded. The non-retained proteins were eluted using buffer C+30 mM imidazole. The bound complexes were finally eluted with buffer C+300 mM imidazole and loaded on SDS–PAGEs as shown in Fig. 5 . All full gels are presented in Supplementary Fig. 3 . Crystallization Initial crystallization conditions were identified using the High Throughput Crystallization platform at EMBL Grenoble (embl.fr/htxlab). Crystals were grown by the hanging-drop vapour diffusion method. Purified protein was diluted to 1.25 mg ml −1 in Tris-HCl 5 mM pH 8.0 containing 0.5 mM of reduced and oxidized glutathione and combined with crystallization solution (12% dioxane) in a 3:1 ratio. Native crystals were harvested, swept through cryoprotection solution (Tris-HCl 5 mM pH 8.0, 12% dioxane, 0.5 mM GSH/GSSG and 25% glycerol) and then plunge-frozen in liquid nitrogen. Data collection and refinement Data from native crystals were collected on the ESRF microfocus beamline ID23-EH2 (ref. 18 ) at 0.873 Å in a gaseous nitrogen cryostream at 100 K. Data were collected using a helical trajectory to distribute radiation damage throughout a larger area of the crystal. Crystals were derivatized by soaking native crystals in 2 mM ethyl mercury thiosalicylate for 2 min, followed by back-soaking into cryoprotection solution and freezing in liquid nitrogen. From the Matthews coefficient, eight protomers were expected in the asymmetric unit. Eight Hg sites were thus identified by SIRAS with SHELXD [19] using a resolution cutoff of 4.8 Å and 800 cycles. Initial sites were then refined in SHARP [20] to 5 Å, yielding an interpretable electron density map and Phasing Powers of 1.15 (isomorphous) for centric reflections, Phasing Powers of 1.18/1.38 (anomalous/isomorphous) for acentric reflections, R cullis of 0.764 (isomorphous) for centric and R cullis of 0.774/0.784 (anomalous/isomorphous) for acentric reflections and Figure of Merit of 0.42/0.37 (acentric/centric). Solvent flattening was performed with PIRATE [20] , a Free-R set was selected in thin shells with SFTOOLS, and an initial model was automatically built in BUCCANEER [21] . This partial model was used to identify the non-crystallographic symmetry operators within the asymmetric unit, which were then used for solvent flattening and non-crystallographic symmetry density averaging in RESOLVE [22] . The model was then improved by multiple rounds of manual model building in COOT [23] followed by refinement in BUSTER with TLS refinement. TLS groups were chosen automatically by BUSTER. Electron density for the majority of the protein construct was of excellent quality, although high-temperature factors were observed at the N-terminus, C-terminal helix and the hairpin loop between residues Pro836 and Gly840. Indeed, the electron density in subunits D, E, F, G and H for this loop was poor and residues 837–839 were therefore omitted from chains F, G and H. Similarly, the density for the C-terminal helix was of good quality in subunit A, but poor for the remaining subunits, especially towards Glu883. However, in subunit E, broken and poorly defined helical density extended further and was modelled as residues Lys887–Ile894, but interpretation of this region should be performed with caution because of the low quality of the electron density. In subunit H, residues Gly885 to Asp896 were ordered and visible, probably because this segment makes crystal contacts with subunit C and F. The final model has a clash score of 1.87 and Ramachandran values (computed with PROCHECK [24] ) of 91.5% core, 8.5% allowed, 0.0% generously allowed and 0.0% disallowed. Data collection and refinement statistics are shown in Supplementary Table 2 . Y2H analysis and protoplasts assays For the Y2H analysis, yeast strains (AH109 and Y187) were transformed by the LiAc method [3] . The Y2H analysis was performed after mating of yeast from the two strains. Interactions were assessed using an HIS3 test, where HIS3 activity resulting from protein–protein interactions is detected by the restoration of growth in the absence of histidine. To do so, OD 600nm were measured during the exponential growth phase in a base medium (SD-Leu/Trp) with or without histidine. For the protoplasts assays, Arabidopsis thaliana (Columbia) seeds were germinated in pots containing Pro-Mix soil and grown at 20°C under constant illumination. Leaves were harvested from 3 to 5-week-old plants and used for protoplast isolation as described previously [11] . Transient expression assays then were carried out either in protoplasts obtained from arf7 mutant leaves (for testing wild-type and mutant ARF7 activity) or from wild-type (for testing wild-type and mutant IAA17/19 activity) containing a single copy DR5:GUS auxin-responsive reporter gene as described [25] . Protoplasts were assayed in absence and presence of 10 mM IAA and quantitative GUS assays were carried out as previously described [25] . In all transfection assays, the 35S:CAT gene (chloramphenicol acetyltransferase, mock) was used in place of the ARF or IAA effector genes as control for the amount of effector plasmid DNA (10 μg) introduced into protoplasts. Statistical significance of the results was tested using the non-parametric Mann–Whitney U -test performed with R ( www.r-project.org ). Accession codes : Coordinates and structure factors of III/IV ARF5 domain have been deposited in the Protein Data Bank under accession code 4CHK . How to cite this article: Nanao, M. H. et al. Structural basis for oligomerization of auxin transcriptional regulators. Nat. Commun. 5:3617 doi: 10.1038/ncomms4617 (2014).